Ligand-induced structural changes in the cyclic nucleotide-modulated potassium channel MloK1 Cyclic nucleotide-modulated ion channels are important for signal transduction and pacemaking in eukaryotes. The molecular determinants of ligand gating in these channels are still unknown, mainly because of a lack of direct structural information. Here we report ligand-induced conformational changes in full-length MloK1, a cyclic nucleotide-modulated potassium channel from the bacterium Mesorhizobium loti , analysed by electron crystallography and atomic force microscopy. Upon cAMP binding, the cyclic nucleotide-binding domains move vertically towards the membrane, and directly contact the S1–S4 voltage sensor domains. This is accompanied by a significant shift and tilt of the voltage sensor domain helices. In both states, the inner pore-lining helices are in an ‘open’ conformation. We propose a mechanism in which ligand binding can favour pore opening via a direct interaction between the cyclic nucleotide-binding domains and voltage sensors. This offers a simple mechanistic hypothesis for the coupling between ligand gating and voltage sensing in eukaryotic HCN channels. Cyclic nucleotide-modulated ion channels play a crucial role in signal transduction and pacemaking in eukaryotes by coupling changes in the levels of the intracellular signalling molecules, cyclic AMP or cyclic GMP, to changes in the ionic flux through the pore of the channel [1] , [2] , [3] . Members of this family include the cyclic nucleotide-gated channels (CNG), which are transducers in the olfactory and visual sensory system [2] , [4] , and the hyperpolarization-activated and cyclic nucleotide-gated channels (HCN) involved in pacemaker activity and resting potential regulation in the heart and brain [1] , [3] , [5] . Topologically, HCN channels are part of the voltage-gated ion channel family. They are tetrameric, with each monomer containing six transmembrane helices (S1–S6), of which the first four helices (S1–S4) form a voltage sensor domain (VSD). Helices S5 and S6 from the four subunits form a single ion-conducting pore in the centre of the tetrameric complex. In addition, CNG and HCN channels have a cyclic nucleotide-binding domain (CNBD) at the carboxy terminus of each monomer. These domains are thought to undergo conformational changes that activate the channel upon cAMP or cGMP binding [4] . The CNBDs are connected to the pore via conserved C-linker domains, which are believed to provide the functional coupling between ligand binding and channel opening [6] . The structures of the isolated CNBD/C-linker regions in liganded form from several HCN channels have been determined using X-ray crystallography [7] , [8] , [9] , [10] , [11] . The isolated CNBDs in the three-dimensional (3D) crystals were arranged in tetramers connected via the C-linker regions, which seemed to establish all contacts between the subunits [4] , [12] . The structures of CNBDs (without C-linkers) in both cAMP-bound and cAMP-free states were determined by X-ray and NMR [13] , [14] , [15] only from a prokaryotic homologue of these channels, MloK1 (also called MlotiK1) from Mesorhizobium loti [16] . The isolated MloK1 CNBDs did not form tetramers in these studies, probably because of the absence of C-linkers and transmembrane domains [15] , [17] . Of all cyclic nucleotide-modulated channels, the only available X-ray structure is that of the MloK1 transmembrane domains [18] . MloK1 functions as a cyclic nucleotide-modulated K + channel despite the presence of an unusually short C-linker containing only ~20 instead of the typical ~80 amino acids [13] , [16] . As expected, the VSDs resolved in the MloK1 transmembrane structure were found in a similar conformation as the voltage-gated K + channel Kv1.2, and the pore region was very similar to that of all other K + channels [18] . The helix bundle gate appeared to be closed and the CNBDs were not resolved in this structure. At present, it is not known whether the MloK1 S1–S4 domain is a functional voltage sensor, since the S4 helix of MloK1 has only two of the six to seven positively charged residues found in other voltage-sensitive channels, and voltage-sensing properties of MloK1 have not yet been reported. The intact, full-length cyclic nucleotide-modulated channel MloK1, has been studied by transmission electron microscopy (EM) as single particles and reconstituted into two-dimensional (2D) crystals, resulting in a 16-Å-resolution 3D model of the structure in the presence of cAMP [19] . Despite its low resolution, this EM analysis showed four CNBDs that make no contacts with each other, arranged with fourfold symmetry in the intact channel. In support of this finding, an atomic force microscopy (AFM) study on 2D crystals of an MloK1-mutant channel also resolved four separate CNBDs in the presence of cAMP. In the absence of cAMP, however, the four CNBDs were coalesced into an unstructured blob that extended about 17 Å away from the membrane [20] . The low resolution and surface topography restriction made it impossible to interpret the molecular mechanisms underlying these observations. Thus, a higher-resolution 3D structure of a full-length cyclic nucleotide-modulated channel in the presence and absence of ligand is needed to gain insight into the mechanism of channel opening upon ligand binding. Here we present the 3D structures of lipid membrane-reconstituted and 2D-crystallized full-length MloK1 in the presence and absence of cAMP determined by cryo-EM of vitrified membranes. For both structures, in presence and absence of cAMP, the densities of the voltage sensor helices (S1–S4) are in good agreement with the X-ray structure of the transmembrane region [18] while the pore helices of our structures suggest a wider opening at the S6 helix bundle. The cAMP-free CNBDs are positioned away from the membrane, but upon ligand binding, these domains approach the membrane and form an intra-subunit interaction with the S1 helix and an inter-subunit interaction with the VSD of the adjacent subunit. Comparison of the two structures indicates that upon cAMP binding the CNBDs approach the membrane vertically by 3 Å, which is accompanied by a rearrangement in the S1–S4 helices and only a small twist of the S6 helices at the bundle opening. The movement of the CNBDs towards the membrane upon ligand binding within the full-length channel was further confirmed by time-resolved AFM topography measurements. A mechanism for ligand gating of cyclic nucleotide-modulated channels is proposed based on the observed conformational changes and the S6 helix bundle conformation. Projection maps of MloK1 2D crystals Well-ordered, large 2D crystals of MloK1 were obtained in the presence and absence of cAMP ( Supplementary Fig. 1a,b ) by mixing detergent-solubilized MloK1 protein with lipids, followed by slow removal of the detergent by dialysis. Liganded MloK1 crystals were grown in 200 μM cAMP conditions, and ligand-free MloK1 crystals were grown by continuously dialyzing for 10 days in cAMP-free buffer. The successful removal of cAMP during the dialysis was verified by analysis of the cAMP content of the ligand-free crystals, reporting that over 97% of the MloK1 molecules were ligand free (see Methods). The cryo-EM images of the plunge-frozen vitrified crystals produced projection maps in good agreement with the Kv1.2 and MloK1 X-ray models [18] , [21] . The grid preparationin conditions were similar to those employed by Clayton et al. [22] ( Supplementary Fig. 1c,d ). In the 2D maps from vitrified crystals grown in both presence and absence of cAMP, MloK1 tetramers are arranged with p 42 1 2 crystal symmetry. The screw-axis symmetry of this crystal form places adjacent MloK1 tetramers in opposite orientations relative to the membrane plane ( Fig. 1b ). These maps showed the MloK1 tetramers to interact with adjacent tetramers via the putative VSDs, while the densities corresponding to the CNBD are outside the membrane plane ( Fig. 1b and Supplementary Fig. 1e ). Differences in the 2D projection maps between the cAMP-free and cAMP-bound conformations indicate rearrangements of the CNBDs, as well as movements of the peripheral regions of the channel, the VSDs ( Supplementary Fig. 1f ). 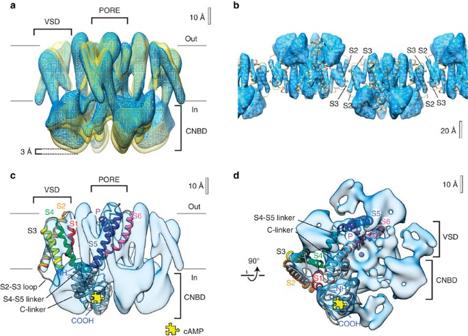Figure 1: 3D cryo-EM maps reveal MloK1 conformations in the presence and absence of cAMP. (a) Superimposed density maps of cAMP-bound (mesh, blue) and cAMP-free (solid, yellow) forms of MloK1. The membrane region as well as the intra- and extracellular sides (labels in and out) are indicated. The channel without ligand is ~3 Å longer than its cAMP-bound counterpart. An equivalent isocontour level was used for both structures. (b) The protein–protein contacts between adjacent, oppositely oriented, cAMP-bound MloK1 tetramers in the 2D crystals are established via the S2 and S3 helices of the VSDs. The model of cAMP-bound MloK1 (brown) is overlapped on the cryo-EM map, which is displayed as raw data without the resolution limitation to 7 × 7 × 12 Å. (c) Density map of MloK1 in the presence of cAMP (blue) shown from the membrane plane, and (d) shown from the intracellular side. A fitted atomistic structure is threaded through one of the subunits. The yellow jigsaw puzzle piece marks the location of the cAMP-binding site; K+and/or Ba+ions are depicted in purple. Atomistic fitting of the 3D maps was performed using a homology model for MloK1 based on the X-ray structure of the transmembrane region (PDB ID 2ZD9 (ref.18)) and the X-ray structure of CNBD in the presence of cAMP (PDB ID 3CL1 (ref.14)). Figure 1: 3D cryo-EM maps reveal MloK1 conformations in the presence and absence of cAMP. ( a ) Superimposed density maps of cAMP-bound (mesh, blue) and cAMP-free (solid, yellow) forms of MloK1. The membrane region as well as the intra- and extracellular sides (labels in and out) are indicated. The channel without ligand is ~3 Å longer than its cAMP-bound counterpart. An equivalent isocontour level was used for both structures. ( b ) The protein–protein contacts between adjacent, oppositely oriented, cAMP-bound MloK1 tetramers in the 2D crystals are established via the S2 and S3 helices of the VSDs. The model of cAMP-bound MloK1 (brown) is overlapped on the cryo-EM map, which is displayed as raw data without the resolution limitation to 7 × 7 × 12 Å. ( c ) Density map of MloK1 in the presence of cAMP (blue) shown from the membrane plane, and ( d ) shown from the intracellular side. A fitted atomistic structure is threaded through one of the subunits. The yellow jigsaw puzzle piece marks the location of the cAMP-binding site; K + and/or Ba + ions are depicted in purple. Atomistic fitting of the 3D maps was performed using a homology model for MloK1 based on the X-ray structure of the transmembrane region (PDB ID 2ZD9 (ref. 18 )) and the X-ray structure of CNBD in the presence of cAMP (PDB ID 3CL1 (ref. 14 )). Full size image Architecture of MloK1 from 3D maps To gain insight into the conformational changes of the entire channel upon cAMP binding, we determined the 3D structures of the membrane-embedded full-length MloK1 protein in the presence and absence of cAMP by electron crystallography. For this, we performed cryo-EM imaging of up to 45°-tilted 2D crystals followed by 3D merging with 2dx (refs 23 , 24 ). This resulted in two 3D data sets that have comparable resolution (7 Å resolution in the membrane plane and 12 Å resolution in the vertical direction) and completeness statistics ( Table 1 , Fig. 1a and Supplementary Fig. 2 ). The MloK1 tetramers in both maps have similar architecture, the expected pore on the fourfold symmetry axis, long densities corresponding to the expected six transmembrane helices per monomer and globular densities corresponding to the CNBDs located below the helices ( Fig. 1 ). An immediately obvious difference between the two maps with and without cAMP is their height difference: the liganded MloK1 is more compact and shorter than the ligand-free MloK1 by about 3 Å ( Fig. 1a ). Table 1 Crystallographic data and statistics. Full size table Precise alignment is required to compare the two cryo-EM maps with one another and with the X-ray structure fragments available for MloK1. To exclude a bias in the z direction due to crystal contacts, we aligned the two maps to each other based on cross-correlation maximization of the transmembrane parts alone ( Figs 1a and 2a ), and docked the X-ray structure of the transmembrane part of MloK1 (PDB ID 2ZD9 (ref. 18 )) into them using Chimera [25] ( Fig. 2b–e ). In both maps, the disposition and packing of the S1–S4 helices as well as the selectivity filter and top portion of the pore region correspond very well to the X-ray data of MloK1 and other voltage-gated channel structures [18] , [21] , [26] ( Fig. 2b ). The crystal contacts of adjacent oppositely oriented tetramers are established by helices S2 and S3 of each subunit ( Fig. 1b ). 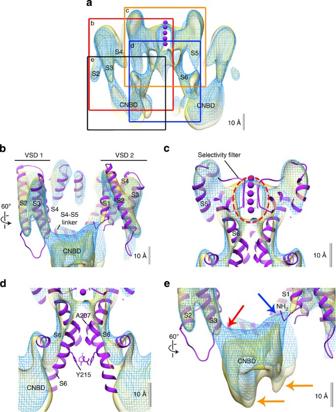Figure 2: The architecture of MloK1. (a) Cross-section through the superimposed cryo-EM maps; the regions of interest (ROI) indicated by the frames are shown in (b–e). MloK1 with cAMP: mesh, blue; MloK1 without cAMP: solid, yellow. The K+ions (purple) inaas well as the ribbon models shown inb–eare from the X-ray structure (PDB ID 2ZD9, purple) and fitted to the cryo-EM map of MloK1 without ligand. (b) Detailed view of the VSDs shows that the X-ray structure agrees with the densities of the cryo-EM maps of MloK1. The tilt of helix S2 with respect to the X-ray structure is evident. (c) Detailed view of the selectivity filter region. The ion densities determined in both cryo-EM maps (red dashed ellipse) are in the selectivity filter region; their positions correspond well to the X-ray structure. (d) Detailed view of the intracellular pore permeation pathway region. Both maps of MloK1 show a significantly wider opening at the helix bundle crossing than the X-ray structure. Residues that form the inner helix bundle crossing (A207) and a constriction region from the X-ray structure (Y215)18are shown as sticks for the X-ray structure. These are clearly outside the cryo-EM maps. (e) Detailed view of the CNBD–VSD interaction region. Upon binding of cAMP, the CNBD undergoes conformational changes resulting in a 3-Å shift towards the lipid bilayer (orange arrows), establishing an interaction of the CNBDs with helix S1 of the same monomer (blue arrow) and helix S3 (red arrow) of the adjacent monomer. Figure 2: The architecture of MloK1. ( a ) Cross-section through the superimposed cryo-EM maps; the regions of interest (ROI) indicated by the frames are shown in ( b – e ). MloK1 with cAMP: mesh, blue; MloK1 without cAMP: solid, yellow. The K + ions (purple) in a as well as the ribbon models shown in b – e are from the X-ray structure (PDB ID 2ZD9, purple) and fitted to the cryo-EM map of MloK1 without ligand. ( b ) Detailed view of the VSDs shows that the X-ray structure agrees with the densities of the cryo-EM maps of MloK1. The tilt of helix S2 with respect to the X-ray structure is evident. ( c ) Detailed view of the selectivity filter region. The ion densities determined in both cryo-EM maps (red dashed ellipse) are in the selectivity filter region; their positions correspond well to the X-ray structure. ( d ) Detailed view of the intracellular pore permeation pathway region. Both maps of MloK1 show a significantly wider opening at the helix bundle crossing than the X-ray structure. Residues that form the inner helix bundle crossing (A207) and a constriction region from the X-ray structure (Y215) [18] are shown as sticks for the X-ray structure. These are clearly outside the cryo-EM maps. ( e ) Detailed view of the CNBD–VSD interaction region. Upon binding of cAMP, the CNBD undergoes conformational changes resulting in a 3-Å shift towards the lipid bilayer (orange arrows), establishing an interaction of the CNBDs with helix S1 of the same monomer (blue arrow) and helix S3 (red arrow) of the adjacent monomer. Full size image The long S6 helices in both EM maps displayed a wider pore opening at the presumed S6 helix crossing than that seen in the MloK1 X-ray structure ( Fig. 2d ). At the level of the presumed helix bundle closure (A207), the pore is ~3 Å wider than that found in the X-ray structure of MloK1. The conformation of the S6 helices in both our EM maps corresponds more closely to that of the X-ray structure of Kv1.2 (at V406), an open pore ( Supplementary Fig. 3 ). The central location of the selectivity filter region showed a large elliptic density, which we attributed to a partial occupancy with K + or other ions (for example, Ba 2+ ) present in the buffer ( Fig. 2c ). In both maps, the long S6 helices are connected to four individually resolved CNBD densities, which can be well docked with the X-ray-determined CNBD structure [14] . In the presence of cAMP, the CNBDs were found in direct contact with the VSD domains and thus abutting the surface of the lipid membrane, while in the absence of cAMP, the CNBDs were seen ~3 Å below this surface. The cAMP-bound CNBD thereby interacts not only with the VSD of its own subunit via the S1 helix but also with the VSD of the adjacent subunit in the same tetramer via the S3 helix ( Fig. 2e ). Structural differences between cAMP-bound and -free MloK1 The alignment of the two maps highlighted significant differences in the CNBDs and the VSD helices between the ligand-free and the liganded MloK1 structures. To better visualize these differences induced in the MloK1 channel by cAMP binding, we constructed atomic models of the full-length channel in the presence and absence of cAMP by flexible model fitting to the cryo-EM maps, starting with the X-ray structures of MloK1 (PDB ID 2ZD9) and isolated CNBDs (PDB ID 3CL1; Figs 1b–d and 3 , Supplementary Movies 1–6 ). 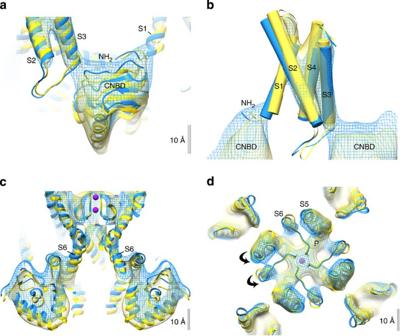Figure 3: Structural changes in MloK1 upon cAMP binding. 3D atomistic models are fitted to the maps of the cAMP-bound (mesh, blue) and cAMP-free (solid, yellow) MloK1 structures. (a) Side view of the CNBD region. Upon ligand binding, CNBDs interacts with the N-terminal region of its own monomer’s S1 helix and the S3 helix of its neighbour. (b) The VSD rearrangement viewed from the side. Helices are shown as cylinders. (c) Cross-section through the transmembrane pore and CNBD regions. (d) Extracellular view on inner helices S5 and S6, which twist slightly counter-clockwise on ligand binding. Figure 3: Structural changes in MloK1 upon cAMP binding. 3D atomistic models are fitted to the maps of the cAMP-bound (mesh, blue) and cAMP-free (solid, yellow) MloK1 structures. ( a ) Side view of the CNBD region. Upon ligand binding, CNBDs interacts with the N-terminal region of its own monomer’s S1 helix and the S3 helix of its neighbour. ( b ) The VSD rearrangement viewed from the side. Helices are shown as cylinders. ( c ) Cross-section through the transmembrane pore and CNBD regions. ( d ) Extracellular view on inner helices S5 and S6, which twist slightly counter-clockwise on ligand binding. Full size image The most prominent change upon cAMP binding is a movement of the MloK1 CNBDs towards the membrane surface that vertically shortens the protein by ~3 Å ( Figs 1a and 2e ). The CNBD structure determined by X-ray crystallography (PDB ID 3CL1) [14] could be docked into the obtained EM maps ( Fig. 3a ). Our structures therefore allow detailed conclusions about the disposition of the CNBDs relative to the membrane parts. However, a higher-resolution cryo-EM analysis will be required to discern conformational changes within the CNBDs upon ligand binding. Comparison of the VSDs from the ligand-free and liganded MloK1 structures and models showed differences in the arrangement of helices S1–S4 ( Fig. 3b ). In the presence of cAMP, and thus while in contact with the CNBDs, all four helices were tilted relative to their more vertical orientation in the absence of ligand. In the presence of cAMP, the largest relative tilts with respect to the central axis of the channel were observed for helix S1 (9°) and helix S2 (6.5°). The linkers connecting helices S4 and S5, believed to play a role in channel gating in other voltage-gated channels, are displaced towards the extracellular side by 1–2 Å in liganded MloK1 ( Supplementary Movies 1 ). The observation of conformational changes of the VSDs following liganding of the CNBDs provides direct evidence of coupling between ligand binding and voltage gating in HCN channels, as further discussed below. We next examined whether there is a change in the pore-opening diameter between the ligand-free and liganded MloK1 structures and models. Inspection of the protein cross-section from the extracellular to the intracellular side shows a small extracellular funnel, the selectivity filter, the S6 helix bundle crossing, the central cavity and an intracellular chamber ( Supplementary Fig. 4 ). The pore helices S6, which are connected to the CNBDs by short (~20 amino acids) C-linkers, are found in very similar positions in both models ( Fig. 3c ). The pore opening at the lower end of the S6 helices (Y215) located between the central cavity and the intracellular chamber has a diameter of 8.5–10 Å ( Fig. 3c and Supplementary Fig. 4b ). Thus, for a hydrated potassium ion of a diameter of ~5.6 Å (ref. 27 ), the opening at the lower end of the S6 helices is always sufficiently wide to allow the passage into the central cavity, regardless of whether cAMP is bound or not. Comparison of the two maps and models further shows that upon ligand binding, helices S5 and S6 are twisted slightly counter-clockwise from their original positions ( Fig. 3d , Supplementary Movies 1–3 ). At the present resolution, the cryo-EM maps do not resolve the state of the S4 helix (3 10 versus α-helical [18] ), nor the changes in the selectivity filter conformation necessary to stop ionic conduction through the pore. Conformational changes in MloK1 imaged with AFM To obtain an independent assessment of the ligand-induced conformational changes in MloK1, we imaged both the liganded and the ligand-free MloK1 2D crystals with AFM. Surface topography recordings by AFM showed the MloK1 2D crystals to be monolayered with an average height in the presence of cAMP of 11.2±0.3 (mean±s.d.) nm and in the absence of cAMP of 11.1±0.4 nm ( Supplementary Fig. 5 ). Individual CNBDs were resolved on the surface of the wild-type MloK1 in topographs recorded in the presence of cAMP showing a left-handed windmill structure in raw data and in average topography ( Fig. 4a , left), while they assembled into a single featureless protrusion in cAMP-free conditions ( Fig. 4a , right). This rearrangement of the CNBDs is accompanied by a height increase of 1.5 nm ( Fig. 4b ). Qualitatively, the increase in height in the ligand-free MloK1 molecules is consistent with the cryo-EM observations but the measured height is much larger. However, the loss of resolution in the AFM images (the transition from a well-resolved tetramer to a featureless protrusion) upon perfusing the ligand out of the sample places some uncertainty on the meaning of the height measured in these conditions. We thus hypothesize that this height is not the effective conformational change undergone in the channel upon ligand removal, but it is a consequence of the CNBDs detaching away from the membrane plane and thus becoming more mobile and more prone to interacting with the AFM cantilever tip. This is also consistent with our previous observation that in the overview images ( Supplementary Fig. 5 ), where there is less tip–sample interaction, the height difference between the crystals in the presence and absence of cAMP is within the error of the measurement and thus much smaller than that measured in the zoomed-in view, where there is more tip–sample interaction ( Fig. 4a ). 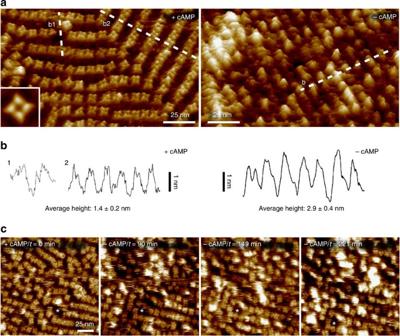Figure 4: AFM analysis of MloK1 in the presence and absence of cAMP. (a) High-resolution AFM topographs of MloK1. In the cAMP-bound state (left), each subunit of the tetrameric channels is well resolved on each single molecule. The four CNBDs were arranged in a left-handed windmill (inset: average). In the cAMP-free state (right), sub-molecular details could not be resolved and the tetramer is contoured as a single protrusion of variable height and appearance. (b) Height profile analysis of MloK1 molecules along the dashed lines ina. In the +cAMP conformation (left), the channels protruded 1.4±0.2 (mean±s.d.) nm (n=50) from the membrane. In absence of ligand (right), MloK1 protruded 2.9±0.4 nm (n=50). A lattice defect was exploited to ensure that the lower protrusion height of the +cAMP conformation was not underestimated owing to the dense molecule packing (height profile b1). (c) Time-lapse AFM of MloK1 channels undergoing the conformational change from cAMP-bound to -unbound state. MloK1 channels were imaged in the presence of 50 μM cAMP (t=0) after which the AFM fluid cell was extensively rinsed with cAMP-free buffer. After incubation time of 90 min, first single MloK1 channels lost their characteristic fourfold symmetric windmill structure and changed into a shapeless protrusion of increased height, and their number increased with time. The asterisks in the four image panels indicate the same membrane position. Figure 4: AFM analysis of MloK1 in the presence and absence of cAMP. ( a ) High-resolution AFM topographs of MloK1. In the cAMP-bound state (left), each subunit of the tetrameric channels is well resolved on each single molecule. The four CNBDs were arranged in a left-handed windmill (inset: average). In the cAMP-free state (right), sub-molecular details could not be resolved and the tetramer is contoured as a single protrusion of variable height and appearance. ( b ) Height profile analysis of MloK1 molecules along the dashed lines in a . In the +cAMP conformation (left), the channels protruded 1.4±0.2 (mean±s.d.) nm ( n =50) from the membrane. In absence of ligand (right), MloK1 protruded 2.9±0.4 nm ( n =50). A lattice defect was exploited to ensure that the lower protrusion height of the +cAMP conformation was not underestimated owing to the dense molecule packing (height profile b1). ( c ) Time-lapse AFM of MloK1 channels undergoing the conformational change from cAMP-bound to -unbound state. MloK1 channels were imaged in the presence of 50 μM cAMP ( t =0) after which the AFM fluid cell was extensively rinsed with cAMP-free buffer. After incubation time of 90 min, first single MloK1 channels lost their characteristic fourfold symmetric windmill structure and changed into a shapeless protrusion of increased height, and their number increased with time. The asterisks in the four image panels indicate the same membrane position. Full size image Furthermore, to ascertain that the changes in CNBDs we observed in the ligand-free crystals are indeed due to ligand removal, we performed time-lapse imaging experiments on the same membrane region while removing cAMP from the AFM fluid cell. Individual MloK1 tetramers underwent conformational changes within a few hours, after which CNBDs revealed an increased height as observed under static conditions ( Fig. 4a ), and could no longer be individually resolved by AFM ( Fig. 4c ). Thus, the occurrence of the conformational change is slow, consistent with previous reports of difficulty in removing the ligand from the binding pocket and obtaining a ligand-free CNBD [28] , [29] . It is important to note that even after 221 min of imaging in the absence of ligand, there are still some well-resolved tetramers that presumably have not yet lost all the ligands, a good internal control that the conformational changes we observe happen at the level of the individual molecules and are not due to AFM-tip–sample interactions. We 2D-crystallized MloK1, a cyclic nucleotide-modulated potassium channel, in the presence and absence of its ligand, cAMP. Cryo-EM imaging of fully hydrated and plunge-frozen samples produced 3D maps at 7 Å resolution in the membrane plane and 12 Å resolution in the vertical direction to which atomic structure models based on the X-ray structures of the isolated transmembrane regions and CNBDs of MloK1 were fitted. A mechanism of channel gating upon cyclic nucleotide binding can be formulated from the observed differences between the two models in the presence and absence of cAMP ( Fig. 5 ). By comparing the two models ( Fig. 5a ) aligned by their selectivity filter as a point of reference, we observed that upon cAMP binding to the CNBDs, the CNBDs approach the lipid membrane and establish contact with the VSDs that shift towards the CNBDs and their helices tilt in the membrane ( Fig. 3b and Supplementary Movies 1–3 ). These conformational changes should favour the opening of the channel pore. However, as indicated by the cryo-EM maps, these domain movements do not lead to any detectable diameter changes either at the level of the Y215 in the cavity or at the lower end of the S6 helices (A207, commonly referred to as the helix bundle crossing). At both levels, our map shows sufficiently wide openings to allow ion permeation, with significantly larger diameters than in the crystal structure of MloK1. 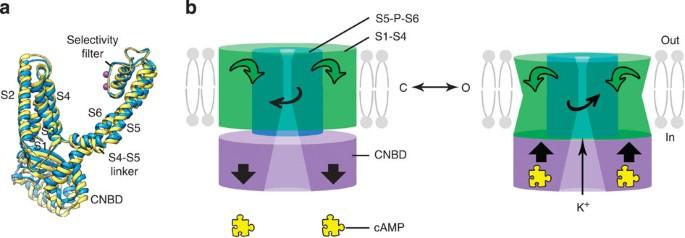Figure 5: Mechanism of MloK1 gating with cAMP. (a) The modelled individual subunits of MloK1 in the cAMP-bound (blue) and cAMP-free (yellow) structures are shown, aligned to the selectivity filters. (b) Proposed mechanism based on the alignment shown ina. Left: without cAMP, right: with bound cAMP (symbolized by the yellow jigsaw puzzle piece). cAMP binding leads to CNBDs (purple cylinder) to move 3 Å towards the membrane, while VSDs (green cylinder) move towards the CNBDs and tilt in lipid bilayer. In parallel, the S5-P-S6 core (blue cylinder) twists slightly in a counter-clockwise (CCW) direction when seen from the extracellular side. This is reversed when cAMP dissociates (left). C/O indicate the closed/open channel configurations. Figure 5: Mechanism of MloK1 gating with cAMP. ( a ) The modelled individual subunits of MloK1 in the cAMP-bound (blue) and cAMP-free (yellow) structures are shown, aligned to the selectivity filters. ( b ) Proposed mechanism based on the alignment shown in a . Left: without cAMP, right: with bound cAMP (symbolized by the yellow jigsaw puzzle piece). cAMP binding leads to CNBDs (purple cylinder) to move 3 Å towards the membrane, while VSDs (green cylinder) move towards the CNBDs and tilt in lipid bilayer. In parallel, the S5-P-S6 core (blue cylinder) twists slightly in a counter-clockwise (CCW) direction when seen from the extracellular side. This is reversed when cAMP dissociates (left). C/O indicate the closed/open channel configurations. Full size image Our data suggest only a very small twist of helices S5 and S6 ( Fig. 3d , Supplementary Movie 2 ). Such small movements near the C terminus of S6 with no pore diameter changes are not in agreement with channel gating at the helix bundle crossing, as observed for KcsA [30] , [31] , [32] , and proposed for voltage-gated channels such as Shaker and Kv1.2 (refs 21 , 33 , 34 ), including HCN-type channels [35] , [36] . Furthermore, the central cavity and lower intracellular chamber of both our MloK1 cryo-EM structures are wider than those in the X-ray structure of MloK1 (ref. 18 ) and have a diameter of 8.5–10 Å, allowing the passage of a hydrated K + ion ( Supplementary Fig. 4b ). The bundle-crossing gate is thus ‘open’ in both ligand-free and liganded conformations, and the helix bundle-crossing opening for both channel forms is larger than that in the X-ray model, suggesting that these channels do not gate at the bundle crossing. An alternative is that the MloK1 channels gate at the selectivity filter. It is possible that the conformational changes occurring in the channel following cAMP binding lead to subtle changes in the selectivity filter (sufficient to restrict or allow permeation). Such changes, as for example, a transition from a KcsA-like collapsed selectivity filter that does not allow K + permeation to a conductive selectivity filter, is unlikely to be captured in our cryo-EM analysis at the current resolution [37] . This type of selectivity filter gating was shown to be involved in C-type inactivation [38] , [39] and also be the major gating mechanism in several ligand-gated ion channels, such as CNG, SK, BK and MthK channels [40] , [41] , [42] , [43] . It appears unlikely that the crystal packing would allow conformational changes at the VSDs, while restricting changes near the channel pore, keeping it in the same state, either open or closed, regardless of whether the ligand is bound or not [44] . Thus, higher-resolution structural data of both channel forms are necessary to pinpoint the location of the gate in MloK1. The cryo-EM structures presented here provide new insight into the arrangement of the CNBDs in the context of the full-length channel in the presence and absence of ligand. In the non-liganded state, these domains are separated from the transmembrane-spanning portions by 3 Å, and make no contact with each other, in agreement with earlier reports [11] , [19] . In the presence of cAMP, however, the CNBDs make direct contact with the membrane and the voltage sensors from both the adjacent and the same subunit, suggesting a simple mechanism for the previously observed coupling between ligand gating and voltage gating in eukaryotic HCN channels [3] , [45] , [46] . The contact of one liganded CNBD to two VSDs (one from the same and the other from an adjacent subunit within the same channel tetramer, as shown in Fig. 2e ) also suggests a way to achieve cooperativity in ligand gating. Eukaryotic CNG and HCN channels are known to display cooperativity in ligand gating [47] , [48] , [49] , [50] . While MloK1 seems to exhibit no ligand-binding cooperativity [28] , [29] , the functional data available for MloK1 are not sufficiently sensitive to determine whether there is cooperativity in ligand gating [13] , [16] . To the best of our knowledge, our study provides the first structural indication that CNBDs and voltage sensors interact directly, although this was proposed recently for HCN channels based on functional assays [51] . Our structures show that in the presence of cAMP, the VSDs are slightly lower in the membrane and their helices are tilted. This finding is in agreement with the observation that cAMP binding in HCN channels lowers the activation voltage. Different mechanistic models have been proposed to describe the movement of the S4 helix and its relation to the other helices in the VSDs of voltage-gated potassium channels [18] , [52] , [53] , [54] , [55] . Of these models, our findings correlate best with the S4 motion in the ‘transporter’-like model, which comprises a tilt and rotation of the S4 helix, accompanied by a 2–3-Å movement [54] . A direct interaction between CNBDs and VSDs also explains why the CNBDs of the tetrameric MloK1 were only resolved in AFM images when cAMP was present, in our work on the wild-type MloK1 as well as in a mutant with lower apparent affinity for cAMP [20] . Under conditions where CNBDs are coupled to the VSDs and thus more restricted in mobility, the AFM is able to contour the CNBDs with nice detail. In the absence of cAMP, the CNBDs lose contact with the VSDs, as shown by cryo-EM, and are thus more mobile so that individual CNBDs could no longer be resolved by AFM. Thus, the protrusion height difference of 1.5 nm (1.7 nm in the mutant [20] ) between the ligand-free and liganded conformations observed by AFM may not reflect a conformational change of that amplitude but corroborates the uncoupling of the CNBDs from the transmembrane portions. Moreover, the in situ time-lapse AFM experiment allowed us to observe the coexistence of both morphologies, clearly indicating that they are two realistic conformations that the channel achieves during gating. In summary, we report the 3D structures of a cyclic nucleotide-modulated potassium channel in the presence and absence of ligand, which allowed us to formulate a mechanism of channel gating upon ligand binding ( Fig. 5b ). We provide structural evidence for direct interaction between the ligand-binding domains and the VSDs during channel gating. Furthermore, based on similar inner pore entrance conformations, we suggest that the channel may not gate at the bundle crossing. MloK1 expression and 2D crystallization Intact, full-length, cyclic nucleotide-modulated potassium channel MloK1 was expressed and purified as described [16] , [19] , with minor modifications. Transformed Escherichia coli cells (BL21(DE3)) containing a C-terminally hexahistidine-tagged MloK1 construct were grown in L-broth at 37 °C. Expression was induced with 0.2 mg ml −1 anhydrotetracycline for 2 h at an OD 600 of 0.7. Cells were pelleted and lysed by sonication. Membrane proteins were solubilized by adding 1.2% n -decyl-β- D -maltopyranoside (Anatrace) to the solubilization buffer (295 mM NaCl, 5 mM KCl, 20 mM Tris–HCl pH 8.0, 10% glycerol, 1 mM phenylmethylsulphonyl fluoride, 0.2 mM cAMP) and incubating for 2.5 h at 4 °C. Extracted MloK1 was purified in 295 mM NaCl, 5 mM KCl, 20 mM Tris–HCl pH 8.0, 10% glycerol, 1 mM phenylmethylsulphonyl fluoride, 40/500 mM (wash/elution) imidazole, 0.2% n -decyl-β- D -maltopyranoside, 0.2 mM cAMP (purification buffer) by Co 2+ -affinity chromatography. To maintain the integrity and function of MloK1, 0.2 mM cAMP (Fluka) was present throughout the purification process. Purified MloK1 was monodisperse as judged by transmission EM imaging. The purified protein in detergent had a tendency to aggregate in the absence of ligand [16] . Pure, detergent-solubilized MloK1 in purification buffer was mixed with E. coli polar lipid extract (Avanti Polar Lipids) at a lipid-to-protein ratio of 0.8–1.0 and dialyzed against detergent-free buffer (20 mM KCl, 20 mM Tris–HCl pH 7.6, 1 mM BaCl 2 , 1 mM EDTA) with and without 0.2 mM cAMP. Protein was 2D crystallized in dialysis buttons for 5–10 days (in buffer with cAMP ligand) or 10 days (in buffer without cAMP ligand) at 37 °C, whereby the dialysis buffer was exchanged every other day. Determination of the bound cAMP After extensive dialysis under crystallization conditions at 37 °C for up to 12 days (buffer-dialysis-volume ratio of ~3,000, several buffer changes), 30 μl of dialysed MloK1 2D crystal sample was digested with 100 μg ml −1 proteinase K (Sigma-Aldrich P2308) with a supplement of 2 mM CaCl 2 at 37 °C for 15 h and centrifuged at 12,000 g at 4 °C for 15 min. SDS–polyacrylamide gel electrophoretic analysis confirmed the absence of any MloK1 protein after proteolysis. Liquid chromatography/mass spectrometry (LC/MS) quantification of the total content of cAMP in the digested sample reported a concentration of less than 0.5 μM cAMP after dialysis. Considering the MloK1 input protein concentration for 2D crystallization of 1 mg ml −1 or 20 μM MloK1, and the LC/MS-determined final cAMP concentration of less than 0.5 μM, the calculated concentration of unliganded MloK1 protein at chemical equilibrium was therefore determined to be higher than 19.5 μM, corresponding to more than 97% of the MloK1 protein being unliganded. Cryo-EM and structure determination MloK1 2D crystal samples in buffer solution with or without cAMP were applied to glow-discharged, thin carbon film-coated copper EM grids. Samples were adsorbed for 1 min in a humid atmosphere. Afterwards, the grids were blotted for 3.5 s and vitrified, without the addition of cryoprotectant, by plunging them into liquid nitrogen-cooled liquid ethane using an FEI Vitrobot MK4 (Vitrobot, Maastricht Instruments). The frozen grids were transferred into a Philips CM200 FEG or a FEI Polara microscope, operated at an acceleration voltage of 200 and 300 kV, respectively, and a nominal magnification of × 50,000–60,000. Low electron dose images were recorded on Kodak SO163 film using a defocus range of 500–2500, nm. Micrographs were checked by optical diffraction, and promising micrographs were digitized on a Heidelberg Primescan D7100 drum scanner with a step size of 5 μm (1 or 0.83 Å per pixel at the specimen level). Digitized images were processed with the 2dx software package ( http://2dx.org [23] , [24] , [56] , [57] ), which is based on the MRC software [58] . Within 2dx, images were corrected for crystal disorder by three rounds of unbending, without the use of any external reference such as generated by MAKETRAN. Defocus and astigmatism were determined by CTFFIND3 (ref. 59 ). The tilt geometry of individual crystals was determined from CTF variations across the image, refined based on lattice distortions and further refined by comparing the single images to the merged 3D data set. 3D merging was done with 2dx_merge, using ORIGTILT [58] , and lattice lines were interpolated with LATLINEK [60] . The Quality Evaluation statistics was reported by 2dx for the 7 × 12 Å 2 resolution-limited data set. A final 3D volume was calculated within 2dx with the CCP4 software package [61] and visualized using Chimera [25] . The validity of the p 42 1 2 screw-axis assignment to the 2D crystals was visible in the absence of forbidden reflections in calculated power spectra of individual images, and verified by 3D processing the entire data set assuming p 4 symmetry, in order to test for any structural differences between the up- and down-oriented tetramers. Care was taken to include images with the correct crystal handedness in correspondence to the grid orientation in the microscope. Albeit at lower resolution, this p 4 processing produced consistently the same conformations for the up- and down-oriented tetramers for both the liganded and unliganded forms, therefore excluding any structural bias from a crystal support film. Flexible model fitting to Cryo-EM maps A starting model was built for the transmembrane part of MloK1 (residues 7–228) from the crystal structure PDB ID 2ZD9 (ref. 18 ), and for the CNBD (residues 229–349) from the crystal structure PDB ID 3CL1 (ref. 14 ). The two structures were placed in the EM density and combined using the program Coot [62] . A first tetrameric model was produced by rigid-body fitting of four copies of this monomer into the density using Chimera [25] . The real-space refinement program DireX [63] was used to fit the structure into the cryo-EM map, applying a B-factor of 200 Å 2 parallel and 450 Å 2 perpendicular to the membrane plane. These B-factors were optimized to best match the point-spread function of the EM density map as calculated by 2dx. A simple Babinet bulk solvent model with k sol =0.6 and B sol =350 Å 2 was used. A mask was applied to avoid artifacts from the periodicity of the 2D protein crystal. The mask was generated as a 30-Å-resolution density map computed from the starting model, and its edges were then steepened with the apply-cos-mapping tool, which is a part of DireX, using 0.25 and 0.15 as upper and lower threshold values, respectively. The four monomers were restrained by non-crystallographic symmetry (NCS) restraints, which keep the monomer structures similar but not identical to each other, with an average root mean squared deviation (r.m.s.d.) of 0.4 Å. We modelled two barium ions; their positions within the channel were maintained by 14 distance restraints to nearby amino-acid side chains. The model was refined into the EM map using 500 steps of DireX refinement. Deformable elastic network restraints were defined between randomly chosen atoms that were within 3–15 Å in the starting structure and separated by no more than 30 amino acids in the sequence, yielding 20,686 restraints, which is twice the number of atoms in the model. Deformable elastic network restraints within α-helices and β-sheets were set to be twice as strong as within loop regions. A cross-validation approach was used to identify the optimally fitted model and to prevent overfitting [64] . In brief, only Fourier components of the cryo-EM maps up to a resolution of 7 Å were used for fitting, while reflections from the ‘free’ interval 5–7 Å were used for validation. For this, the cross-correlation coefficient, C free , was calculated between the model density map and the cryo-EM density map, both of which were band-pass filtered to the ‘free’ interval, thus containing information that had not been used for fitting. The same starting model was fitted into both density maps, that is, for the cAMP-bound and cAMP-free states, and the same set of DireX parameters were used. During the refinement, the C free value for the cAMP-free case increased from 0.081 to 0.142 and the C work value increased from 0.794 to 0.833. For the cAMP-bound case, the C free value increased from 0.048 to 0.154 and the C work value increased from 0.688 to 0.827. The refined models were further optimized using CNS [65] with 1,000 steps of Cartesian dynamics at a temperature of 40 K followed by 300 minimization steps. For both dynamics and minimization, all hydrogen atoms were added to the model and electrostatic interactions were only used between backbone atoms to improve the hydrogen-bonding network. In addition, statistical Ramachandran restraints were used to improve the backbone dihedral angles. As the conformation of the CNBDs in the final models for both conformations was quite similar to each other with an r.m.s.d. of 0.8 Å, we generated a second starting model as a control. This was built from the same transmembrane part (residues 7–228) from crystal structure PDB ID 2ZD9 (ref. 18 ) as before, but the CNBDs (residues 229–349) were replaced by the open NMR CNBD structure PDB ID 2KXL [15] determined in absence of cAMP. Refinements from this second starting model, using the same DireX parameters as the previous refinements, resulted in final refined structures with rather large r.m.s.d. from the starting model of 7.8 and 7.3 Å in the presence and absence of cAMP, respectively. The large conformational changes occurring during the refinements and the lower C free values of 0.114 and 0.087 in the presence and absence of cAMP, respectively, indicated that these final models from the second starting model were of much lower quality than with the first starting model. An analysis of the internal conformations of the CNBDs was therefore not feasible with the current cryo-EM data. Difference map Difference maps were calculated for the 2D projection maps of MloK1 with and without cAMP, limited to 7 Å resolution. The alignment of the individual projection maps was achieved using the common phase origin of the p42 1 2 symmetry gained from the MRC program ALLSPACE [66] and refined by MRC program ORIGTILT [58] , all within the 2dx software. The merged projection maps were scaled to [0,1], and a raw difference map was calculated by subtraction of one map from the other. To determine the significance of the differences, we calculated the variations within the individual projection maps, in a similar manner as done before [67] . To this end, we empirically determined the variations across the two conformations by randomly splitting images from both conformations into two sets, averaging the images from both sets and calculating the corresponding difference map. Repeated application of this procedure resulted in a large number of difference maps, which were then averaged to produce a general variation map. Differences between conformations with and without cAMP were only considered to be significant if they exceeded those present in the variation map. The final result was visualized as a heat map using Matplotlib. Atomic force microscopy MloK1 2D crystal preparations (as above) were adsorbed on freshly cleaved mica at a protein concentration of 0.1 mg ml −1 in 10 mM Tris, pH 7.4, 150 mM KCl, 3 mM EDTA, and in case of cAMP-bound crystals containing additional 50 μM cAMP (Sigma-Aldrich). After 20 min incubation, the sample was rinsed carefully with 10 mM Tris, pH 7.4, 150 mM KCl buffer±cAMP (as indicated) to remove non-adsorbed membrane crystals. Membranes were imaged in contact-mode AFM using a Nanoscope E system (Bruker, Santa Barbara, CA, USA) equipped with a 160-μm scanner (J-scanner), a fluid cell and OMCL TR400PSA cantilevers (Olympus, Tokyo, Japan) with a nominal spring constants of 80 pN nm −1 . The measurements were performed in buffer solution and at ambient temperature and pressure. Imaging forces were minimized to ~100 pN. Images were acquired at scanning frequencies of 4–7 Hz and optimized proportional and integral gain parameters were used. A more detailed description of AFM data acquisition can be found in ref. 68 . For time-lapse AFM experiments, the sample was washed thoroughly by exchanging 10 times the volume of the fluid cell with cAMP-free buffer, and the very same MloK1 membrane patch was continuously imaged. Accession codes : The cryo-EM volumes are available at the EM Data Bank, accession codes EMD-2526 (with cAMP) and EMD-2527 (without cAMP). The atomic models are available at the Protein Data Bank, accession codes 4CHV (with cAMP) and 4CHW (without cAMP). The raw cryo-EM image data used for calculating the maps reported here, together with the employed 2dx processing parameters, are available as public data set at the http://www.ebi.ac.uk/~ardan/aspera/em-aspera-demo.html under accession number 10006. How to cite this article: Kowal, J. et al. Ligand-induced structural changes in the cyclic nucleotide-modulated potassium channel MloK1. Nat. Commun. 5:3106 doi: 10.1038/ncomms4106 (2014).